Bio-barcode gel assay for microRNA MicroRNA has been identified as a potential biomarker because expression level of microRNA is correlated with various cancers. Its detection at low concentrations would be highly beneficial for cancer diagnosis. Here, we develop a new type of a DNA-modified gold nanoparticle-based bio-barcode assay that uses a conventional gel electrophoresis platform and potassium cyanide chemistry and show this assay can detect microRNA at aM levels without enzymatic amplification. It is also shown that single-base-mismatched microRNA can be differentiated from perfectly matched microRNA and the multiplexed detection of various combinations of microRNA sequences is possible with this approach. Finally, differently expressed microRNA levels are selectively detected from cancer cells using the bio-barcode gel assay, and the results are compared with conventional polymerase chain reaction-based results. The method and results shown herein pave the way for practical use of a conventional gel electrophoresis for detecting biomolecules of interest even at aM level without polymerase chain reaction amplification. Various microRNAs (miRNAs), 19- to 25-nucleotide-long small non-coding RNAs, act as regulators in biological processes such as gene expression, tumorigenesis, cell proliferation and apoptosis, via hybridization with target messenger RNA [1] . miRNA has been implicated in cancer of abnormal complex genetic diseases through their function as oncogenes or tumour suppressors [2] , [3] , and it will be highly beneficial to detect multiple miRNA sequences at a very low concentration for understanding and diagnosing cancers in reliable fashion [4] , [5] . Although many new types of miRNA-detection methods have been developed, polymerase chain reaction (PCR) based methods have been dominantly used for detecting an ultra-low amount of miRNA convincingly [5] , [6] , [7] . Although utterly sensitive, the PCR has limitations including its complex, expensive, time-consuming, and labour-intensive procedure [8] , [9] . Especially for the multiplexed detection of short targets with a similar length such as miRNA, it is impossible or very difficult to differentiate them in the gel image, and more importantly, short primer sequences and low temperature are used for the PCR process for short targets due to the low melting temperature for short primer hybridization. This can cause the limited primer hybridization efficiency, nonspecific hybridization and erroneous results. In the case of the real-time PCR for miRNA (typically, hairpin-containing miRNA precursors are used in this case), primer design and complicated normalization and optimization techniques are required and very challenging in many cases [10] . Further, many newly developed methods are typically based on highly complicated, untested and non-conventional setups, and this significantly prohibits the widespread use of these methods. This includes nanoparticle-based bio-barcode assay that detects protein and DNA with ultrahigh sensitivity [11] , [12] , [13] , [14] , [15] , and although shown highly sensitive and versatile, this method is yet to be widely used partly because of the use of a non-conventional light-scattering assay platform. Further, it is very difficult to reliably and sensitively detect 19- to 25-nucleotide-long miRNA targets because miRNA is easily degradable by RNase [16] . In this regard, the bio-barcode approach that detects a barcode DNA that is a surrogate for a miRNA target could be beneficial. Here, we develop a bio-barcode gel (bio-BaGel) assay for detecting an ultra-low amount of miRNA with a conventional gel electrophoresis platform without enzymatic amplification. In this assay, two different types of probes are designed and used; the barcode and magnetic probes. The assay is named as the bio-barcode assay because an artificially designed DNA represents each miRNA target sequence in a way that a specific barcode label represents a specific product. Instead of directly detecting miRNA, the final assay signal is obtained from the amount of barcode DNA. In this way, one can significantly amplify the detection signal without any enzymatic amplification because a number of barcode DNA strands can be modified to each barcode probe (gold nanoparticle (AuNP), in this case). In our approach, a barcode DNA has two regions; one region that can capture target miRNA and the other region with a varying length of the encoding sequence. Depending on the length of the encoding region, double-stranded barcode DNA bands appear differently in the gel electrophoresis results. The other probe is the magnetic probe, and can be formed by modifying the other-half target miRNA complements. After sandwich-capturing target miRNA with the barcode and magnetic probes, magnetic probe-captured barcode probes can be readily separated by a magnetic field. Finally, we find that potassium cyanide (KCN) can dissolve AuNPs to completely release barcode DNA in a very short time and further amplify the detection signal intensity during the gel electrophoresis of double-helix barcode DNA (dx-barcode DNA) sequences. The bio-BaGel assay offers a straightforward detection signal amplification strategy on a conventional gel electrophoresis platform. The detection dynamic range of the assay spans from aM to nM, and the multiplexed detection of several different miRNA targets in one sample is also possible using the bio-BaGel method. We further show the bio-BaGel assay is able to detect varying miRNA levels from breast and lung cancer cells with high sensitivity and selectivity. We expect this conventional gel and KCN-dissolution-based bio-BaGel assay to be widely utilized for the sensitive identification and quantification of various miRNA sequences. Design of DNA sequences for probes We selected three different miRNA sequences (miR-205, miR-21 and miR-155), which are known to play a major role in cancer [17] , [18] . For the detection of these miRNAs, we designed DNA sequences for barcode and magnetic particles in a way that many barcode DNA strands were modified to an AuNP and target miRNA could be sandwich-captured by barcode and magnetic probes ( Fig. 1a and Supplementary Tables 1 and 2 ). For the multiplexed detection, we inserted extra bases (4, 9 and 14 bases for miR-205, miR-21 and miR-155, respectively) to each barcode DNA sequence. The different length of each barcode DNA provides the separation among these three different barcode DNA sequences due to the different mobility during the electrophoresis on a non-denaturing polyacrylamide gel [19] . 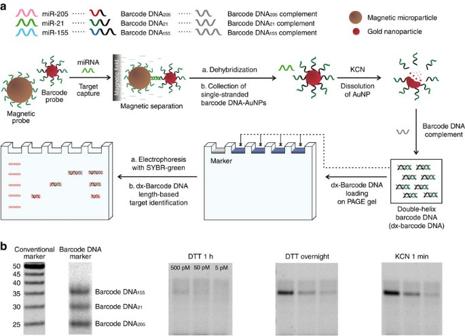Figure 1: Bio-barcode gel assay and KCN-based barcode DNA release. (a) The schematic diagram of the bio-barcode gel assay for miRNA. (b) Barcode DNA release and detection after 20 mM DTT or 50 mM KCN treatment. The concentration of gold nanoparticle (AuNP) probes was varied from 500 pM to 5 pM. The left two gel images show the conventional marker bands and our barcode reference bands (25mer, 30mer and 35mer), respectively. The right three gel-images are the barcode DNA gel assay results after 1 h and overnight DTT treatment and 1 min KCN treatment, respectively. Figure 1: Bio-barcode gel assay and KCN-based barcode DNA release. ( a ) The schematic diagram of the bio-barcode gel assay for miRNA. ( b ) Barcode DNA release and detection after 20 mM DTT or 50 mM KCN treatment. The concentration of gold nanoparticle (AuNP) probes was varied from 500 pM to 5 pM. The left two gel images show the conventional marker bands and our barcode reference bands (25mer, 30mer and 35mer), respectively. The right three gel-images are the barcode DNA gel assay results after 1 h and overnight DTT treatment and 1 min KCN treatment, respectively. Full size image Bio-BaGel assay In a typical experiment, 100 μl of target miRNA solution was mixed with barcode and magnetic probes (10 μl of 500 pM barcode probe solution and 10 μl of 15 pM magnetic probe solution) in a microtube, and the mixture was incubated at 95 °C (above the melting temperature) for 3 min. For the negative control experiment, 100 μl of 100 pM non-complementary miRNA was used, and this background miRNA was added to all the samples. The resulting solution was then incubated at room temperature for 1 h with vigorous shaking. After the incubation, target miRNA-sandwiched barcode and magnetic probe complexes were separated by applying the magnetic field for 2 min. After discarding the supernatant, the pellet was dispersed in 15 μl of deionized (DI) water and incubated at 95 °C for 5 min to break up the complexes via DNA de-hybridization. The magnetic field was re-applied to remove the magnetic probes and recover the barcode probes. We then added 350 mM (final concentration of 50 mM) KCN to dissolve AuNPs to efficiently recover barcode DNA strands and the resulting solution was incubated for 1 min with heating ( Fig. 1b and Supplementary Fig. 1 ) [20] . It should be noted that dithiothreitol (DTT) is typically used to detach the thiolated DNAs from AuNPs through ligand exchanges [21] . We compared KCN and DTT methods, and the results show that KCN is a much more efficient agent for releasing barcode DNA strands from AuNPs with respect to time and amount of DNA ( Fig. 1b ). When KCN was treated for 1 min for 5–500 pM barcode probe solution, the gel band was stronger than the DTT case even with overnight incubation. To check the applicability of KCN chemistry to DNA-modified silver nanoparticles (40-nm AgNPs), we prepared the DNA-modified AgNP probes with barcode DNA 205 using the same salt-aging method with AuNP probe preparation. For the DNA-striping process, we used DTT and KCN for 1 min and overnight, respectively. In the gel image for 1-min treatment, KCN is more efficient than DTT reagent to detach DNA from surfaces of AgNP with respect to signal intensity and assay time. However, the difference is less dramatic, especially for overnight case, than AuNPs ( Supplementary Fig. 2 ). This could be mainly because DNA–AgNPs are less stable than DNA–AuNPs. Thiol–AgNP interaction can be much more easily broken than thiol–AuNP complex because the binding energy of thiol-Ag is weaker than that of thiol-Au [22] . AgNP is chemically less stable and induces the cytotoxicity through mitochondrial dysfunction, induction of reactive oxygen species and DNA damage [23] while the cytotoxicity of AuNPs, compared with AgNPs, is negligible [24] , [25] . For these reasons, DNA–AuNPs are more reliable and versatile materials than DNA–AgNPs in our case. Next, to decode KCN-recovered barcode DNA and to detect barcode DNA with double-stranded-DNA-intercalating fluorescent dyes on gel, 5 μl of 10 μM barcode DNA complements was added to form dx-barcode DNA and 3.97 μl of 2 M NaCl, and the resulting solution was incubated at 4 °C for 30 min (ref. 26 ). These dx-barcode DNA strands were then loaded on the well of 12% non-denaturing polyacrylamide gel to identify and quantify miRNA via the detection of dx-barcode DNA. After the electrophoresis at 300 V for ~2 h, the gel was stained by SYBR Green I (1:10,000 diluted solution) for 30 min and was washed with DI water. Finally, the gel was imaged by the gel document system with UV lamp at 306 nm wavelength and ~1,500 ms exposure time ( Fig. 2 ). 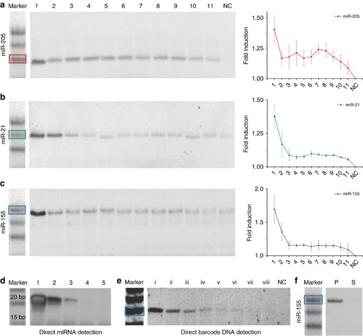Figure 2: Bio-BaGel assay results for a single miRNA target. The bio-BaGel assay results for miR-205 (a), miR-21 (b) and miR-155 (c) targets from 10 nM to 1 aM target concentrations with a negative control (NC) band (lanes 1–11: 10 nM, 1 nM, 100 pM, 10 pM, 1 pM, 100 fM, 10 fM, 1 fM, 100 aM, 10 aM and 1 aM). The highlighted gel marker region is the position of the corresponding double-helix barcode DNA strands. The graph shows the average fold-induction values for the gel band intensity for each target concentration, normalized with the negative control band intensity. The error bars are the s.d. obtained from four independent experiments for each case. (d) Direct miRNA-detection results (lanes 1–5: 10 nM, 1 nM, 100 pM, 10 pM and 1 pM). (e) Direct barcode DNA-detection results (lane i–viii: 1 pmole, 100 fmole, 10 fmole, 1 fmole, 100 amole, 10 amole, 1 amole and 100 zmole). (f) Single-base-mismatched miRNA-detection results (perfect match (P) and single-base-mismatch (S) miRNA-detection results). Figure 2: Bio-BaGel assay results for a single miRNA target. The bio-BaGel assay results for miR-205 ( a ), miR-21 ( b ) and miR-155 ( c ) targets from 10 nM to 1 aM target concentrations with a negative control (NC) band (lanes 1–11: 10 nM, 1 nM, 100 pM, 10 pM, 1 pM, 100 fM, 10 fM, 1 fM, 100 aM, 10 aM and 1 aM). The highlighted gel marker region is the position of the corresponding double-helix barcode DNA strands. The graph shows the average fold-induction values for the gel band intensity for each target concentration, normalized with the negative control band intensity. The error bars are the s.d. obtained from four independent experiments for each case. ( d ) Direct miRNA-detection results (lanes 1–5: 10 nM, 1 nM, 100 pM, 10 pM and 1 pM). ( e ) Direct barcode DNA-detection results (lane i–viii: 1 pmole, 100 fmole, 10 fmole, 1 fmole, 100 amole, 10 amole, 1 amole and 100 zmole). ( f ) Single-base-mismatched miRNA-detection results (perfect match (P) and single-base-mismatch (S) miRNA-detection results). Full size image Bio-BaGel assay results and analysis for a single target The single miRNA target-detection results for miR-205, miR-21 and miR-155 are shown respectively in Fig. 2a–c . A wide detection range from 1 aM to 10 nM target miRNA solution was examined. Importantly, as low as 1–10 aM target solution was detected with 100 μl sample volume. For each detection target, the position of each dx-barcode DNA matched well with the marker band. From the 1–10 nM target concentration range, a significant increase in gel band intensity was observed. We verified our results by comparing the bio-BaGel assay results to conventional reverse transcription–PCR (RT–PCR) results with the same miRNA target. We detected the target 100 nM, 100 pM, 100 fM and 100 aM miRNA samples (1 μl sample volume) through 30 cycles of the RT–PCR in parallel with our method ( Supplementary Fig. 3a ). For each case, three independent sets of experiments were repeated to obtain the error bars. The overall trends of the fold-induction results from the bio-BaGel and RT–PCR are similar. However, in the case of RT–PCR, it should be noticed that it is difficult or impossible to design the primer and amplify mature miRNA due to the short miRNA length, which can lead to erroneous results [10] , [27] , [28] , [29] , [30] . The negative control band of RT–PCR shows relatively higher signal than that of the bio-BaGel assay. Consequently, the bio-BaGel method could be more straightforward and reliable in detecting short miRNA, especially at very low concentrations than the PCR method. To estimate how much our assay improved the miRNA-detection sensitivity, a conventional gel electrophoresis (12% non-denaturing polyacrylamide gel) assay for the direct detection of miRNA without dx-barcode DNA amplification was performed ( Fig. 2d ). The result shows that 10–100 pM target concentration is the detection limit in this case. To dissect the reason for this improvement in sensitivity, we first quantified the amount of modified barcode DNA strands per AuNP. The fluorophore-labeled barcode DNA strands were liberated into solution by the addition of KCN and quantified by the measurement of fluorescence signal ( Supplementary Fig. 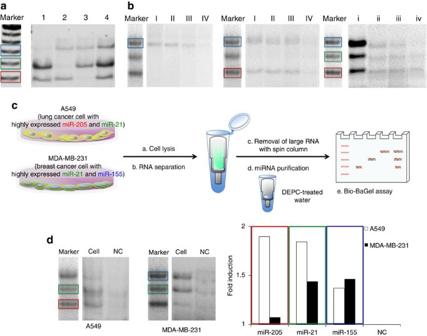Figure 3: Multiplexed miRNA detection. (a,b) The results of multiplexed detections of various combinations of miRNA sequences ((a) lane 1: miR-205 and miR-21, lane 2: miR-205 and miR-155, lane 3: miR-21 and miR-155, lane 4: miR-205, miR-21 and miR-155; (b) lane I– IV: 1 nM, 1 pM, 1 fM and NC and lane i–iv: 30 nM, 300 pM, 300 fM and NC). (c) The schematic diagram of the miRNA detection from two different cancer cell lines with the bio-BaGel assay. (d) The bio-BaGel assay results from MDA-MB-231 and A549 cell lines, respectively. All the experiments were repeated four times for each case. The graph values were normalized by the signal from the negative control. 4 and Supplementary Table 3 ). Approximately 1,500 barcode DNA strands were modified for each 50-nm AuNP, which provides ~1,500-fold amplification for each miRNA-detection event. The number of loaded DNAs per AuNP directly affects signal amplification in our case. Therefore, 50-nm AuNP with larger amount of DNA (~1,466 strands per AuNP) is more appropriate than 20 nm (378 strands per AuNP) and 30 nm (723 strands per AuNP) for the bio-BaGel assay ( Supplementary Fig. 5 and Supplementary Table 4 ) [21] . One can argue the use of even larger AuNPs, but there are limitations for larger AuNPs (>60-nm AuNPs) for the reliable and quantitative bio-BaGel assay results. The preparation and handling of larger AuNPs is much more delicate and difficult in salt-contained buffer solution for bioassay applications [31] . In general, the larger AuNPs are less stable than smaller particles and can easily form aggregates. We also checked the barcode DNA-detection limit with 12% non-denaturing polyacrylamide gel ( Fig. 2e ). The data show that 10 amole (1 pM) barcode DNA can be detected in this case, and this supports that the detection limit for barcode DNA can be one or two orders-of-magnitude better than miRNA detection. We then tested our assay selectivity with single-base-mismatched miRNA sequence for miR-155 ( Fig. 2f ). As shown in the gel image, the bio-BaGel assay can clearly differentiate the single-base-mismatched miRNA from the perfectly matched miRNA (10 nM target concentration for both cases). Multiplexed detection of three different miRNA targets Next, we tested the multiplexing capability of the bio-BaGel assay with three different miRNA targets (miR-205 with 25mer barcode DNA, miR-21 with 30mer barcode DNA and miR-155 with 35mer barcode DNA, respectively). First, various combinations of 10 nM miRNA sequences were detected with the bio-BaGel assay (the added miRNA sequences are shown above the gel image), and the result shows that the assay has a very good selectivity for the miRNA sequences that are present in the samples ( Fig. 3a ). We further performed the multiplexed bio-BaGel assay at much lower target miRNA concentrations. As shown in Fig. 3b for single-, two- and three-target miRNA cases, the results support the high selectivity of this method even at fM miRNA range. Figure 3: Multiplexed miRNA detection. ( a , b ) The results of multiplexed detections of various combinations of miRNA sequences (( a ) lane 1: miR-205 and miR-21, lane 2: miR-205 and miR-155, lane 3: miR-21 and miR-155, lane 4: miR-205, miR-21 and miR-155; ( b ) lane I– IV: 1 nM, 1 pM, 1 fM and NC and lane i–iv: 30 nM, 300 pM, 300 fM and NC). ( c ) The schematic diagram of the miRNA detection from two different cancer cell lines with the bio-BaGel assay. ( d ) The bio-BaGel assay results from MDA-MB-231 and A549 cell lines, respectively. All the experiments were repeated four times for each case. The graph values were normalized by the signal from the negative control. Full size image Multiplexed miRNA detection from cancer cells Finally, to check the usefulness of this assay for biological studies, we applied the bio-BaGel assay to identify the highly expressed miRNA sequences from lung (A549) and breast (MDA-MB-231) cancer cell lines, respectively. The real-time PCR-based results suggest that MDA-MB-231 overexpresses the miR-21 and miR-155 sequences, whereas miR-205 is decreased [32] . Although the miR-205 and miR-21 sequences are increased in A549, miR-155 is decreased [4] , [33] . For the bio-BaGel assay, 80% confluent cells were lysed with a cell lysis buffer that induces the rupture of cell membrane and inactivates RNase. miRNA was then extracted with the miRNA isolation kit (E.Z.N.A miRNA kit, OMEGA bio tek, GA, USA) ( Fig. 3c ). After the miRNA isolation, the extracted miRNA was checked with the UV–vis spectrometer, RT–PCR and the electrophoresis ( Supplementary Figs 6 and 7 ). The bio-BaGel assay results with these cell-extracted miRNA samples are shown in Fig. 3d . Larger amounts of miR-155 and miR-21 and lower amount of miR-205 for MDA-MB-231 cells and larger amounts of miR-21 and miR-205 and lower amount of miR-155 for A549 cells were detected, and the results matched well with the literature results using hairpin-containing miRNA precursors. We confirmed the reproducibility of the detection results for the cell extract samples from four individual experiments. These results validate the usefulness of the bio-BaGel assay for the selective detection of miRNA in biological samples. We also compared our results with the conventional RT–PCR results. In the case of the RT–PCR method, it is impossible to differentiate short miRNA sequences (22 bp for all three miRNA sequences) in the gel image, and, multiplexing three different miRNA targets with the same length in one sample was not possible. For the short targets including miRNA, short primer sequences were used and low temperature was applied for the PCR due to the low melting temperature for primer hybridization. Because of these, primer hybridization efficiency is limited and nonspecific hybridization can occur. However, in the case of the bio-BaGel assay, we were able to perform the multiplexed assay for three different targets because of the use of a synthetic barcode DNA-based surrogate approach. In Supplementary Fig. 7 , the RT–PCR for each target was performed separately to compare the RT–PCR results to the bio-BaGel assay results. When we compared the bio-BaGel assay results for two different cell lines (A549 and MDA-MB-231; Fig. 3d ) with the RT–PCR results ( Supplementary Fig. 7b ), the difference between different miRNA sequences is more distinct in the case of the bio-BaGel assay that requires no primer-based enzymatic amplification. We developed the bio-BaGel assay for the ultrasensitive detection of miRNA and showed that the detection of aM level of miRNA is possible on a conventional gel platform without the use of PCR. This was possible because each nanoparticle carries ~1,500 barcode DNA for a single miRNA-detection event and the detection of artificially designed barcode DNA gives a higher sensitivity than the direct detection of miRNA, which is often unstable. Further, the KCN-based release of barcode DNA from AuNPs is very fast and highly efficient. We rigorously tested the usefulness of the bio-BaGel assay in various target miRNA concentrations (aM to nM), single-base-mismatched sequence discrimination and multiplexed detection. Importantly, the bio-BaGel assay results for the varying miRNA levels of three miRNA sequences from breast and lung cancer cell lines matched well with the real-time PCR-based premature miRNA-detection results from the same cell lines. This is an important step forward considering the RT–PCR for short sequences such as miRNA is often difficult and can generate erroneous results. This conventional gel-based bio-BaGel assay paved ways for the practical and widespread use of the ultrasensitive miRNA-detection method without using the enzymatic amplification techniques, such as PCR and other expensive, complicated setups. DNA-modified magnetic microparticle (MMP) preparation We used amine-functionalized oligonucleotides and 1-μm-carboxylic acid functional group-coated MMPs (Dynabeads MyOne Carboxylic Acid, Invitrogen, NY, USA). After 30-min vortexing, the MMPs (1 ml) were transferred to a new tube. To remove the supernatant, the tube was placed in a magnet for 2 min. The MMPs were then washed twice with 100 mM 2-[ N -morpholino]ethane sulphonic acid (MES) buffer with pH 4.8 and were resuspended in 100 μl of the same buffer. The mixture of 5′-amine-modified oligonucleotides (50 nmol) and 40 μl of 1.25 mM N -ethyl- N ′-[3-dimethylaminopropyl]carbodiimide hydrochloride in 100 mM MES (pH 4.8) was added to washed the MMPs. After 4-h incubation at room temperature, the MMPs were washed three times with 1 ml Tris-Tween-20 (TT) buffer which contained 250 ml of 1 M Tris buffer (pH 8) and 1 ml 10% Tween-20 and diluted to 1,000 ml with distilled water. Finally, DNA-modified MMPs were suspended in 1 ml of Tris-EDTA buffer. For the preparation of Tris-EDTA buffer, 10 ml of 100 mM EDTA (ethylenediaminetetraacetic acid disodium salt) was mixed with 10 ml of 1 M Tris buffer (pH 8), and then this solution was diluted to 1,000 ml with distilled water. Barcode DNA-modified gold nanoparticle preparation Disulphide-protecting group-modified oligonucleotides were reduced by 100 mM DTT to yield free thiolated oligonucleotides. After reducing, excess DTT was removed by NAP-5 column (GE Healthcare, UK). Freshly reduced thiolated oligonucleotides were added to 50-nm gold nanoparticles solution. The mixed solution was placed on an orbital shaker at room temperature overnight. The solution was then adjusted to obtain a final phosphate concentration of 100 mM (pH 7.4) with 0.1% (wt/vol) SDS. After 30-min incubation, the mixed solution was brought to 0.3 M NaCl by the addition of ten aliquots of 1 M NaCl solution and was then incubated at room temperature overnight. The solution was centrifuged (6,000 r.p.m., 15 min), the supernatant was removed and the precipitate was finally redispersed in 0.15 M PBS solution (pH 7.4). Bio-BaGel assay procedures RNase-free materials were used throughout experiments. First, miRNA was dissolved in RNase-free water at a concentration of 100 μM (stock solution). For the preparation of a certain miRNA concentration, the stock miRNA solution was diluted with phosphate-buffered saline solution (10 mM phosphate, 150 mM salt, pH 7.4). In a typical experiment, 10 μl of MMP solution (15 pM) and 10 μl of AuNP solution (500 pM) were brought together in a tube (final volume of 120 μl by adding PBS solution). After 3-min annealing in a 95 °C water bath, the solution was further vortexed and incubated for 1 h. The MMP-target-AuNP complexes were collected by applying a magnetic field, and the supernatant was removed to get rid of unbound free AuNPs and other remnants. The collected MMP-target-AuNP complexes were redispersed in 15 μl of distilled water and incubated in 95 °C water for 2 min to dehybridize the complexes and release AuNP probes from the complexes. The released AuNPs were collected by applying a magnetic field and recovering the supernatant from the solution. Next, 2.5 μl of KCN (350 mM) (Sigma Aldrich, CA, USA) and 5 μl of decoding DNA (10 μM) were added to the released AuNP solution, followed by annealing in a 95 °C water bath for 3 min. KCN completely dissolved AuNPs to fully release barcode DNA, and decoding DNA was hybridized with released barcode DNA to result in double-helix barcode DNA via incubation at room temperature for 30 min, and double-helix barcode DNA was then mixed with 3 μl of DNA-loading dye (glycerol, orange G and xylene cyanol FF). For the multiplexed miRNA detection, target miRNA solution was diluted with PBS buffer to prepare miRNA samples with a concentration range from 30 nM to 3 aM. First, three different MMPs with three different miRNA complements and three AuNP probes with three different miRNA complements were mixed. Then, 100 μl of each miRNA target solution was added to prepare samples with different targets to result in 360 μl of total sample volume. Direct detection of miRNA and barcode DNA For the direct hybridization between miRNA and its complementary DNA, the miRNA solution was diluted to various concentrations, ranging from 10 μM to 10 nM. A volume of 5 μl of diluted miRNA solution was mixed with 5 μl of complementary DNA (100 μM), and salt concentration was adjusted to 150 mM using 2 M NaCl solution. For the direct hybridization between barcode DNA and its complement, the barcode DNA was diluted to various concentrations, ranging from 200 nM to 20 fM. Next, 5 μl of 100 μM decoding DNA (barcode DNA complement) was added to 5 μl of barcode DNA solution, and salt concentration was adjusted to 150 mM using 2 M NaCl solution. Fluorescence measurement To quantify the number of barcode DNA strands per AuNP, Cy3-modified barcode DNA was used to prepare barcode DNA-modified AuNP probes. Then, 10 μl of KCN was mixed with 90 μl of AuNP probes. The fluorescence intensity of released Cy3-modified barcode DNA was measured with a fluorometer (JASCO, MD, USA) at a fixed cell temperature of 25 °C. The excitation wavelength was 480 nm and the emission intensity at 560 nm was used to calculate the number of DNA. The standard curve was obtained using the same DNA with known concentrations. To estimate the enhancement by SYBR Green, SYBR Green solution was diluted with dimethyl sulphoxide (Sigma Aldrich), and 45 μl of diluted SYBR Green solution was mixed with 15 μl of AuNP solution and 10 μl of KCN solution. The total volume of samples without AuNP or KCN was adjusted to 70 μl for all samples by adding distilled water. The excitation and emission wavelengths were 477 nm and 550 nm, respectively, and cell temperature was fixed at 25 °C. Cancer cell culture The MDA-MB-231 (ATCC, Num. HTB-26) and A549 (ATCC, Num. CCL-185) were purchased from American type culture collection. MDA-MB-231, human breast carcinoma cell, was cultured in 10% fetal bovine serum that contains RPMI media (Gibco, Invitrogen, NY, USA) with 100 units per ml penicillin-streptomycin (Gibco, Invitrogen). A549, human lung carcinoma cell, was grown in Dulbecco’s modified Eagle’s medium (Gibco, USA) with 10% fetal bovine serum and antibiotics. All the cell lines were incubated at 37 °C with 5% CO 2 . miRNA isolation from cancer cells We used E.Z.N.A miRNA kit (OMEGA bio tek, GA, USA) for the extraction of miRNA of two different cancer cells (MDA-MB-231 and A549). For cell lysis, we added 1 ml of RNA-Solv reagent into 1 × 10 7 cultured cells grown in a monolayer. The lysate was transferred to a clean 2-ml microcentrifuge tube. After 3-min incubation at room temperature, we added 0.2 ml chloroform to 1 ml lysate-contained RNA-Solv reagent and then vortex it vigorously for 15 s. The mixed solution was incubated on ice for 10 min and centrifuged at 12,000 g at 4 °C for 15 min. The upper aqueous phase was transferred to a new 2-ml microcentrifuge tube. We added 300 μl of 100% ethanol and vortex thoroughly. To remove large RNA, the mixed solution was centrifuged at 10,000 g for 1 min using HiBind RNA mini column. The 1 ml of filtrate was collected and measured. We then added 650 μl of ethanol to the filtrate. For the isolation of miRNA, we used HiBind Micro RNA column. After centrifugation of the mixed solution at 10,000 g for 1 min, HiBind Micro RNA was washed by RNA wash buffer II via centrifugation at 10,000 g for 1 min. After washing, HiBind Micro RNA was transferred to a clean 2-ml microcentrifuge tube, and we added 15 μl of DEPC-treated water and incubated at room temperature for 2 min. Finally, we obtained miRNA through centrifugation at full speed for 1 min. We characterized the miRNA using UV–vis spectrometer and gel electrophoresis and used this miRNA for dx-barcode assay. Polyacrylamide gel electrophoresis To distinguish different dx-barcode DNA seqeunces with 5 bp difference, we used the 12% neutral polyacrylamide gel that consists of 30% acrylamide/Bis solution (Bio-rad, CA, USA), deionized water, 5 × TBE buffer (Sigma Aldrich), APS (Sigma Aldrich) and TEMED (Sigma Aldrich). The dx-barcode DNA mixture with loading dyes (Fermentas, Maryland, USA) was added to each well of a 1.5-mm-thick gel (Galileo Bioscience, MA, USA). To confirm the DNA molecular weight on a gel, we also loaded the 5-bp DNA ladder (Fermentas) to other well. We applied the electric field to gel in tank (Galileo Bioscience, MA, USA) at 300 V for 2.5 h using power supply (Hoefer, MA, USA). After electrophoresis, gel was stained by SYBR Green I (Lonza, NJ, USA) for 30 min and was de-stained by deionized water for 1 min. Finally, gel was imaged using UV light excitation at 306 nm by a gel imager (Corebio, Seoul, South Korea). Statistical analysis We obtained the error bars in the graphs in Fig. 2 from the results of four independent experiments. To obtain the statistical average and standard deviation values, we repeated four experiments for each case and the gel images were analysed with Adobe Photoshop program CS6 (Adobe, CA, USA). We measured the same size of the area at each band using the rectangular marquee tool of the Adobe Photoshop CS6. The measured intensities were normalized by dividing each detection signal value by the negative control signal intensity from the same gel, and the fold-induction value (the ratio between detection signal and noise signal (negative control)) at each target concentration was then obtained. The error bars are the s.d. of the fold-induction-based band intensities after normalization. We also repeated the experiments for the data in Fig. 3 four times. We demonstrated that the results were fairly reproducible. Reverse transcription–PCR (RT–PCR) We designed three different sense and antisense primers for each target miRNA. Three sense primers are primer 1: 5′-TCCTTCATTCC-3′, primer 2: 5′-TAGCTTATCAG-3′, and primer 3: 5′-TTAATGCTAAT-3′. And three antisense primers are r-primer 1: 5′-CAGACTCCGGT-3′, r-primer 2: 5′-TCGGCATCATG-3′, and r-primer 3: 5′-CCCCTATCACG-3′. For RT–PCR, we diluted pure synthetic miRNA at 100 nM, 100 pM, 100 fM, 100 aM, and 100 zM and used the volume of 1 μl. The primers, dNTPs, each miRNA and polymerase were mixed in a PCR tube (total volume: 20 μl) for amplification. We ran 30 cycles of the RT–PCR (2720 Thermal Cycler, Applied Biosystems, CA, USA) and confirmed the amplified oligonucleotides using 12% neutral polyacrylamide gel. We also used two kinds of cell extracts for miRNA detection through the RT–PCR. The RT–PCR experiments for cell extracts were performed using the same procedure as described above. How to cite this article: Lee, H. et al. Bio-barcode gel assay for microRNA. Nat. Commun. 5:3367 doi: 10.1038/ncomms4367 (2014).